Coastal pollution limits pelagic larval dispersal The ecological impact of large coastal human populations on marine ecosystems remains relatively unknown. Here, we examine the population structure of Patiria miniata , the bat star, and correlate genetic distances with a model based on flow rates and proximity to P. miniata populations for the four major stormwater runoff and wastewater effluent sources of the Southern California Bight. We show that overall genetic connectivity is high ( F ST ∼ 0.005); however, multivariate analyses show that genetic structure is highly correlated with anthropogenic inputs. The best models included both stormwater and wastewater variables and explained between 26.55 and 93.69% of the observed structure. Additionally, regressions between allelic richness and distance to sources show that populations near anthropogenic pollution have reduced genetic diversity. Our results indicate that anthropogenic runoff and effluent are acting as barriers to larval dispersal, effectively isolating a high gene flow species that is virtually free of direct human impact. Human beings have impacted every marine ecosystem on earth, and almost half of these systems have been strongly affected by multiple anthropogenic factors [1] . The ecological consequences of anthropogenic impacts have become too large to ignore, and recent efforts have been made to incorporate them into management and conservation strategies [2] , [3] . However, in addition to recognizing humans as the world's most powerful evolutionary force [4] , we have little information on anthropogenic impacts to the evolutionary processes of non-harvested species, such as population connectivity, and this specific information remains a critical missing element in almost all marine conservation [5] , [6] . Over 17 million people, close to 25% of the entire US coastal population [7] , [8] , inhabit the coastal area of the Southern California Bight (SCB), and it represents one of the most affected marine ecosystems in the world [1] . Besides habitat loss and modification, the next largest environmental impact of this urban population is the discharge of contaminants into the ecosystem [7] . The SCB has more than 60 point sources discharging ∼ 4.7 billion liters of effluent per day, with the two largest sources of contaminants being sewage effluent from municipal treatment plants (wastewater) and runoff from highly modified natural river basins (stormwater) [9] . This effluent transports large loads of known and unknown contaminants, including heavy metals, chlorinated hydrocarbons, petroleum hydrocarbons, nutrients and bacteria [7] , and has been shown to be toxic to marine fauna [10] . A wide range of anthropogenic chemicals has been shown to disrupt the hormonal systems of wildlife species and have become a major cause for concern in global efforts to conserve biodiversity [11] . Many of these substances are also known to be toxic to larvae [12] , [13] , [14] . We hypothesized that anthropogenic effluent and runoff and the transported contaminants associated with them are toxic to larvae, therefore affecting marine population connectivity in the SCB by inducing broad-scale larval mortality. To test whether population connectivity was limited by stormwater and wastewater contaminants, we examined the population structure of Patiria miniata , the common bat star, across 16 populations in the SCB. P. miniata is a ubiquitous omnivore found along the subtidal and intertidal west coast of North America. It has a 6–10-week pelagic larval development period, a potential year-round breeding season that may peak in summer [15] , [16] , and has been shown to have both high genetic diversity and high genetic connectivity between populations over 1,000-km apart [17] . Moreover, P. miniata is a non-fished, non-harvested species relatively free from any direct human impact, making it a conservative system to test for human-mediated effects on connectivity. We found stormwater and wastewater to be effective barriers to larval dispersal, reducing gene flow between populations. Furthermore, wastewater (and most likely stormwater) sources effectively lower genetic diversity. Thus, our study suggests a role for human impact in altering larval dispersal. Population connectivity We sequenced 439 individuals at two mitochondrial DNA (mtDNA) genes and genotyped them at seven microsatellite loci (nDNA). 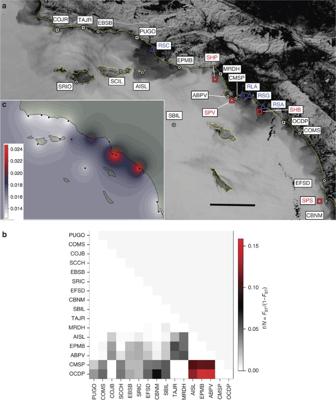Figure 1: Visualization of anthropogenic correlations ofP. miniatapopulation structure. (a) Map and satellite image ofP. miniatapopulation sampling sites highlighting the four wastewater sources (red squares) and the four stormwater sources (blue triangles). The image is a reverse black and white rendering of an image from the NASA MODIS satellite on 1 December 2005 (http://rapidfire.sci.gsfc.nasa.gov/subsets/?subset=AERONET_La_Jolla.2005012.aqua.250m) showing visible sediment from stormwater. White squares represent populations withn<20, whereas white circles are populations withn>20. Each population is also labelled with a four-letter code for reference. Red squares are the locations of wastewater outfalls and blue triangles are the locations of stormwater sources (river mouths). Pollution source abbreviations are RLA, The Los Angeles River; RSA, The Santa Ana River; RSG, The San Gabriel River; SHB, outfall for the Huntington Beach wastewater treatment facility; SHP, Hyperion sewage treatment plant; SPS, outfall for the Point Loma wastewater treatment plant and SPV, outfall for the Rancho Palos Verdes wastewater treatment plant. (b) A heat map colour-coded by pairwise linearizedFSTvalues from the LD mtDNA marker. (c) A Kriging surface interpolation using the average pairwiseFSTvalue for each population averaged across each of the three marker sets. Scale bar, 50 km. As expected, genetic diversity is extremely high ( Table 1 , Supplementary Fig. S1 ) and the overall genetic structure of P. miniata is low, with global F ST values ranging between 0.001 and 0.007 and only one of those values being statistically significant. However, examining pairwise differentiation values among sites showed that there is a distinct geographic pattern to the genetic structure of P. miniata ( Fig. 1 ), and the structure appeared to correlate visually with the major sources of anthropogenic contaminants in the SCB ( Fig. 1 ). Table 1 Genetic diversity of Patiria miniata. Full size table Figure 1: Visualization of anthropogenic correlations of P. miniata population structure. ( a ) Map and satellite image of P. miniata population sampling sites highlighting the four wastewater sources (red squares) and the four stormwater sources (blue triangles). The image is a reverse black and white rendering of an image from the NASA MODIS satellite on 1 December 2005 ( http://rapidfire.sci.gsfc.nasa.gov/subsets/?subset=AERONET_La_Jolla.2005012.aqua.250m ) showing visible sediment from stormwater. White squares represent populations with n <20, whereas white circles are populations with n >20. Each population is also labelled with a four-letter code for reference. Red squares are the locations of wastewater outfalls and blue triangles are the locations of stormwater sources (river mouths). Pollution source abbreviations are RLA, The Los Angeles River; RSA, The Santa Ana River; RSG, The San Gabriel River; SHB, outfall for the Huntington Beach wastewater treatment facility; SHP, Hyperion sewage treatment plant; SPS, outfall for the Point Loma wastewater treatment plant and SPV, outfall for the Rancho Palos Verdes wastewater treatment plant. ( b ) A heat map colour-coded by pairwise linearized F ST values from the LD mtDNA marker. ( c ) A Kriging surface interpolation using the average pairwise F ST value for each population averaged across each of the three marker sets. Scale bar, 50 km. Full size image Anthropogenic effects on genetic structure To specifically test the effects of stormwater and wastewater on genetic structure, we created a simple model based on the average flow rate of the contaminant source and the distance of that source from our sampled populations. That model was then used to create pairwise 'resistance' matrices for all of our populations. We examined how well anthropogenic resistance matrices predicted the pairwise values of genetic structure, connectivity ( F ST ) and differentiation ( D EST ), using single and multiple matrix regression (MMR) frameworks [18] and a distance-based canonical redundancy analysis. Single-variable regression Examining pollution sources in a single-variable framework revealed consistent and significant limitations to gene flow associated with contaminant sources. 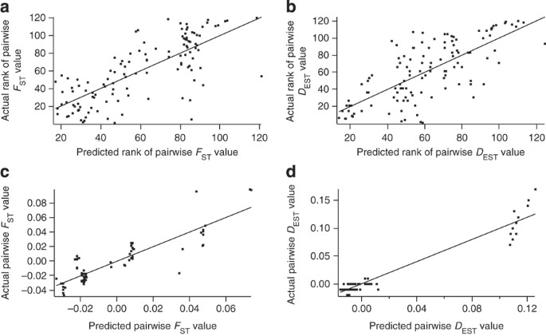Figure 2: Graphs of the best multivariate models using the LD mtDNA loci. (a) Predicted rankFSTversus actualFSTrank using the full population data set.R2=0.5768,P-value<0.0001. (b) Predicted rankDESTversus actualDESTrank, using the full population data set.R2=0.5406,P-value<0.0001. (c) PredictedFSTversus actualFST, using then>20 data subset.R2=0.7621,P-value<0.0001. (d) PredictedDESTversus actualDESTusing then>20 data subset.R2=0.9369,P-value<0.0001. DIST, geographic distance. Overall, several stormwater and wastewater variables have high and significant correlations to several measures of genetic structure using the low diversity (LD) mtDNA locus ( Table 2 , Supplementary Table S2 ). In contrast, no significant predictors were found for the nDNA data sets. Neither geographic distance nor the stormwater input from the Santa Clara River (RSC) was found to be a significant predictor for any data set. Table 2 Single anthropogenic source regression results. Full size table Multivariate regression Expanding models to include more than one predictive variable greatly improved the model fit for all data sets, highlighting the synergistic effect of multiple anthropogenic sources on the genetic structure of P. miniata . 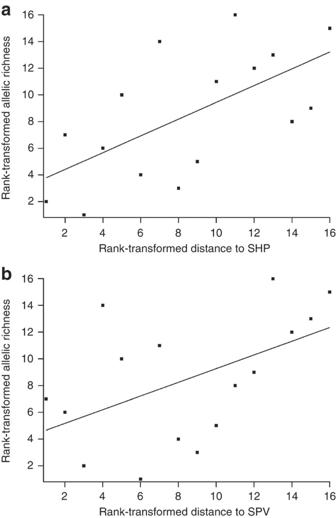Figure 3: Graphs of the two significant predictors of nDNA AR. (a)R2=0.3962,P-value=0.0090 and (b)R2=0.2619,P-value=0.0427. Every top model included both stormwater and wastewater variables ( Table 3 , Supplementary Tables S3–S8 ), indicating that both are important in driving the observed patterns of genetic structure. Although there were significant models predicting nDNA genetic structure, they often had relatively low R 2 values (0.11–0.14) compared with that using mtDNA loci (0.22–0.57). Models predicting genetic structure values using the LD mtDNA marker showed the highest R 2 values (0.54–0.58) and the best fit ( Fig. 2 ). Table 3 Multiple anthropogenic source regression results. Full size table Figure 2: Graphs of the best multivariate models using the LD mtDNA loci. ( a ) Predicted rank F ST versus actual F ST rank using the full population data set. R 2 =0.5768, P -value<0.0001. ( b ) Predicted rank D EST versus actual D EST rank, using the full population data set. R 2 =0.5406, P -value<0.0001. ( c ) Predicted F ST versus actual F ST , using the n >20 data subset. R 2 =0.7621, P -value<0.0001. ( d ) Predicted D EST versus actual D EST using the n >20 data subset. R 2 =0.9369, P -value<0.0001. DIST, geographic distance. Full size image Among stormwater sources, three were present in every top mtDNA model: the Los Angeles River, the San Gabriel River and the Santa Ana River. RSC was included in several models, but was usually nonsignificant. Among all loci, the Hyperion and Palos Verdes sewage outfalls were included in all top models, whereas the Point Loma outfall appears in two of the six models. The Huntington Beach outfall is not included in many models and is often insignificant when it does. This is most likely because of its proximity and spatial autocorrelation with Santa Ana River. Canonical redundancy analysis MMR is one of the better performing methods of evaluating the influence of landscape (seascape) variables on genetic structure; however, it has recently been suggested that the best analytical strategies involve using multiple types of analyses [19] . To this end, we used a distance-based canonical redundancy analysis, that has been shown to have not only relatively low power for detecting effects but also low type-1 error rate [19] , to redo all single variable regressions ( Supplementary Table S9 ) and to test the six top models from the MMR analysis ( Supplementary Table S10 ). The results were nearly identical to the MMR and corroborate our initial findings. Population sampling size and high-diversity genetic markers Despite its ubiquitous nature, P. miniata was rare at some sites, and despite extensive survey, some populations only had 15 individuals sampled. For genetic markers with high mutation rates and especially for species with low levels of genetic structure, under-sampling of populations may lead to inaccurate measures of genetic structure [20] , [21] . To control for this possibility, a subset of the data was reanalyzed using only populations with more than 20 individuals sampled. This data subset represents a balance between increasing the accuracy of our genetic measures while still retaining 11 of the 16 original populations and maintaining sufficient geographic sampling ( Fig. 1 , Supplementary Table S1 ). For all stormwater and wastewater models, R 2 values increased using the subset of well-sampled populations ( Tables 2 and 3 , and Fig. 2 ). In single variable tests, almost all significant variables from the full data set remained significant ( Table 2 , Supplementary Table S2 ). For multivariate models, the top models had increased R 2 values and included fewer variables than top models using the full data set; however, they still included both wastewater and stormwater variables ( Table 3 ). For multivariate models, removing populations, especially those bordering or between anthropogenic inputs, lessened geographic sampling, leading to higher correlations between predictive matrices and therefore less variables in the top models. Using the data subset also decreased the large discrepancy between R 2 values of multivariate models for the two mtDNA loci, demonstrating that under-sampling had a large effect on the genetic structure values from the higher polymorphism marker. In all cases, R 2 values were greater for models using either of the mtDNA markers compared with the nDNA markers. Loss of genetic diversity due to anthropogenic isolation To examine the effects of wastewater and stormwater sources on genetic diversity, rarefied nDNA allelic richness (AR) for each population was regressed to the distance of each population from a single effluent source. There were positive correlations between AR and distance away from every wastewater and stormwater source; however, only two sources had significant relationships ( P <0.05), wastewater sources Hyperion and Palos Verdes ( Fig. 3 ). Figure 3: Graphs of the two significant predictors of nDNA AR. ( a ) R 2 =0.3962, P -value=0.0090 and ( b ) R 2 =0.2619, P -value=0.0427. Full size image Contemporary versus historical effects Examining the relative roles of contemporary and historical seascape effects on genetic connectivity is essential to any seascape genetic study [22] . The stormwater sources examined in this study are also the mouths of natural rivers. Without accurate estimates of historical river outputs, there is no way of separating contemporary anthropogenic influences of increased urban runoff, more consistent outflow and extensive riverbed engineering [7] , from the potential historical effects of natural river flow in these variables. Therefore, a conservative approach was taken and all stormwater variables were treated solely as historic variables, and wastewater variables were treated as the only contemporary anthropogenic variables and examined in an MMR framework. For each measure of population structure, an MMR model using only historic (stormwater) variables was selected by AICc (Akaike information criterion adjusted for small sample sizes) value. The residuals, or unexplained variance, of that model were then used as a response variable in an MMR model using only contemporary (wastewater) variables. This specifically examines whether contemporary variables can explain significant portions of population structure that are unexplained by historic variables. Anthropogenic wastewater variables explained significant amounts of residual variation in three of the six models tested with the full data set and all six models tested with the n >20 subset ( Table 4 ), conclusively showing that contemporary variables have considerable influence on the population connectivity of P. miniata . Table 4 Stormwater residual regression results. Full size table The high and significant correlations of anthropogenic environmental variables with the population structure of P. miniata demonstrate the utility of using a spatially explicit model to examine influences on population connectivity. Single variable and multivariate modelling show that human beings have a profound influence on the population connectivity of a ubiquitous, non-harvested species with high levels of genetic diversity and gene flow. This anthropogenic isolation is most likely caused by larval mortality from the substantial contemporary augmentation of freshwater, particulate and/or pollutant load into the SCB. Most seascape genetic studies have focused on the role of oceanographic factors in determining genetic structure [23] , [24] , [25] , [26] , [27] , [28] . The SCB, however, is an oceanographically unique system with heterogeneous and variable mesoscale eddies influencing short-term circulation and the Southern California Cyclonic Gyre dominating longer term circulation patterns [29] . Ocean-based circulation models for connectivity in the SCB have shown rather stable patterns within single spawning seasons with large amounts of heterogeneity between seasons [30] , and most simulations with larvae in the water column for 30 or more days showed high levels of connectivity between most sites, with a general pattern of mainland sites as sources and the Northern and Southern Channel Islands as sinks [31] . Moreover, a comprehensive seascape genetics study of three separate species in the SCB revealed that oceanographic processes were poor predictors of genetic connectivity and diversity in species with longer pelagic larval durations [32] . Considering the 6–10-week larval development period and year-long breeding season of P. miniata [15] , [16] , oceanographic factors are most likely weak influences on the genetic connectivity and diversity of this species and were subsequently not included in any models. In any study examining anthropogenic effects on evolutionary processes, it is critical to be able to separate historic, natural processes from contemporary anthropogenic ones [22] , [33] . It could be argued that the genetic structure of P. miniata has been shaped historically for thousands of generations by natural rivers. However, several key results from this study point to the anthropogenic nature of the observed effects. The current generalization in landscape genetics is that microsatellites are the best genetic markers suited for studies of contemporary gene flow [22] , [34] , [35] . This is most likely because of the fact that the majority of landscape genetics studies have been on vertebrates and plants in the terrestrial systems [22] in which effective population sizes are small and genetic variation may be difficult to find. However, in an organism with high genetic diversity and a large effective population size, such as P. miniata , this is likely not the case and the crucial factor becomes not the mutation rate of the marker but whether or not there is enough variation within the landscape [36] . Recently isolated populations (<50 generations) that were previously very diverse and well connected will not have time to accumulate much differentiation by mutation, even in fast-evolving markers [37] . Consequently, almost all current spatial genetic information is contained in extant alleles [37] . In fact, most spatial autocorrelation is created over 20–50 generations, and its detectable signal wanes in markers with the highest mutation rates [37] . In these situations, the only evolutionary force acting on allele frequencies in these populations will be genetic drift, which has larger effects on smaller effective population sizes [38] , and has been shown to be rampant in artificially fragmented populations [39] . Therefore, considering the high genetic diversity of P. miniata and previous connectivity [17] , we would expect to see a more pronounced signal of anthropogenic isolation in the mtDNA markers, which have an effective population ∼ 1/4 the size of the nDNA markers [38] . In all population structure models tested, we observed that R 2 values were ∼ 1.5–30 times higher for mtDNA markers relative to nDNA markers ( Tables t2 , t3 , t4 ), although results from nDNA genetic diversity regressions were consistent with anthropogenic isolation ( Fig. 3 ). This indicates that the observed structure is most likely due to the very recent isolation of these previously well-connected populations and not due to a historical pattern of isolation. Wastewater variables also contain valuable information about the temporal scale of the observed gene flow patterns as they are completely contemporary and anthropogenic. Here, we observed wastewater variables in all top multivariate models and high and significant correlations to genetic structure in single variable tests. Distance away from two stormwater sources was also significantly correlated to nDNA genetic diversity ( Fig. 3 ). Moreover, when stormwater variables were treated as historical variables, despite the fact that stormwater runoff has been greatly augmented by urbanization and riverbed civil engineering [7] , wastewater variables still explained significant amounts of variation in genetic structure not explained by 'historic variables' ( Table 4 ). These results strongly suggest that human-mediated inputs have a profound influence on the genetic structure of P. miniata . Finally, RSC is the second largest source of stormwater by volume [24] ; however, it was only significantly correlated to genetic structure in one single-variable test, and that correlation was negative. RSC was also not included in many of the top multivariate models and when it was included, typically it was nonsignificant ( Table 3 ). RSC is the least populated, least urbanized and least modified watershed of the four stormwater sources [40] , and these three factors correlate directly to pollutant and contaminant loading [41] . Thus, we argue that it is contaminant loading and not freshwater river input that drives the significant deviation from panmixia detected in this study. In summary, our results clearly indicate that coastal pollution is limiting the larval dispersal and population connectivity of P. miniata . However, even if the observed effects were purely from historical river input, these results would still have far-reaching implications. This is because both stormwater volume and wastewater volume have increased with the human population of the SCB, augmenting and dwarfing historical natural runoff, especially during dry weather periods [7] . Consequently, the broad, immediate conservation implications of these results would not change; the current paradigm for the incorporation of wastewater and stormwater in ecosystem-based management needs to be rethought. Population genetic methods Microsatellite loci were genotyped according to ref. 17 with the exception of using dye-labelled primers and an ABI 3730XL for genotyping. Two mtDNA loci were sequenced, a tRNA region and part of the cytochrome oxidase subunit I gene (COI) [17] and control region (CR) [42] . The two mtDNA loci were analysed as a LD marker (COI) and as a full mtDNA marker (COI+CR). This was carried out to add more phylogenetic information to the diverse CR loci (268 unique haplotypes). F ST values for mtDNA loci were calculated using the Phi ST estimator of ARLEQUIN [43] . F ST values for microsatellites were calculated using the Phi ST estimator in GenoDive [44] . D EST values were calculated using SMOGD [45] and SPADE [46] . AR was calculated using rarefaction to 15 individuals per population using FSTAT [47] . Seascape genetic methods Shortest sea distance was calculated between every population and each stormwater and wastewater source using Google Earth ( http://earth.google.com ). Distances were then entered into the model: PW=flow×exp(−0.1×distance), where flow is the average daily flow (in millions of gallons per day) of the contaminant source. Effluent plumes are subject to oceanographic conditions. Modelling of plumes is well beyond the scope of this project, so PW was based on a simple function of exponential decay. The coefficient of −0.01 was chosen for simplicity and for the property of decreasing ∼ 100-fold by ∼ 50 km and quickly approaching zero thereafter. This was an attempt to match the approximate distance between adjacent populations. Results were also examined using an alternate PW model, PW=flow/(distance) 3 , approximating volumetric expansion and were similar (data not shown). PW statistics were summed for each pair of populations to create pairwise matrices of 'ecological distance' or 'resistance' for each anthropogenic source. Matrices were analysed in an MMR framework [18] , [33] with F ST and D EST values as dependent values. For the full data set, all matrices, with the exception of full mtDNA values, were rank transformed after examining the residuals of regressions using untransformed data. The n >20 data set was untransformed. Significance was calculated using 10,000 random permutations of matrices. All MMR analyses were performed in the R statistical package [48] using the ecodist package. AICc values were calculated using JMP 8 (SAS). Canonical redundancy analyses were performed in R using package rdaTest with 10,000 permutations used to assess significance. For single-variable tests, all three F ST or all three D EST were combined into one simultaneous test, and whenever geographic distance was found to be significant, it was included in all other variable tests as a covariable. Data Deposition: Coordinates and mtDNA sequence data have been deposited in GenBank under accession numbers codes from JF296310 to JF297187 . How to cite this article: Puritz, J. B. & Toonen, R. J. Coastal pollution limits pelagic larval dispersal. Nat. Commun. 2:226 doi: 10.1038/ncomms1238 (2011).